Made-to-order metal-organic frameworks for trace carbon dioxide removal and air capture Direct air capture is regarded as a plausible alternate approach that, if economically practical, can mitigate the increasing carbon dioxide emissions associated with two of the main carbon polluting sources, namely stationary power plants and transportation. Here we show that metal-organic framework crystal chemistry permits the construction of an isostructural metal-organic framework ( SIFSIX -3-Cu) based on pyrazine/copper(II) two-dimensional periodic 4 4 square grids pillared by silicon hexafluoride anions and thus allows further contraction of the pore system to 3.5 versus 3.84 Å for the parent zinc(II) derivative. This enhances the adsorption energetics and subsequently displays carbon dioxide uptake and selectivity at very low partial pressures relevant to air capture and trace carbon dioxide removal. The resultant SIFSIX- 3-Cu exhibits uniformly distributed adsorption energetics and offers enhanced carbon dioxide physical adsorption properties, uptake and selectivity in highly diluted gas streams, a performance, to the best of our knowledge, unachievable with other classes of porous materials. The amount of carbon dioxide (CO 2 ) in the atmosphere continues to rise and rather rapidly due to unparalleled cumulative CO 2 emissions, provoking the undesirable greenhouse gas effect. Certainly, it is becoming critical to develop economical and practical pathways to reduce the CO 2 emissions; and appropriately prospective routes to address this enduring challenge are considered: (i) CO 2 emission reduction from post-combustion stationary and mobile sources [1] where CO 2 concentration is in the range of 10–15% and (ii) CO 2 removal from air called direct air capture (DAC), which is another alternative option to reduce greenhouse gases emissions in a uniform way globally [1] , [2] , [3] , [4] . Although DAC is relatively more challenging than post-combustion capture, it is recognized that it might be practical, provided that suitable adsorbent combining optimum uptake, kinetics, energetics and CO 2 selectivity is available at trace CO 2 concentration [5] . In addition, efficient and cost-effective removal of trace CO 2 is of prime importance in various key industrial applications pertaining to energy, environment and health. From an industrial perspective, the removal of trace CO 2 from air is a growing area of research and development due to its substantial importance for prepurification of air and particularly when atmospheric air is used during the separation of nitrogen and oxygen. In fact, before air separation using cryogenic distillation or pressure swing adsorption, air must be CO 2 free to avoid (i) blockage of heat-exchange equipment as a result of frozen CO 2 during the liquefaction process [6] , [7] and (ii) adsorbents (for example, zeolites) contamination used for oxygen production by pressure swing adsorption [8] , [9] , [10] . Equally important, alkaline fuel cells require a CO 2 free feedstock of oxygen and hydrogen gases as it is widely recognized that trace amounts of CO 2 (that is, 300 p.p.m.) degrade the electrolyte in alkaline fuel cells [11] . Furthermore, efficient removal of CO 2 at low concentrations is also vital for the proper operation of breathing systems in confined spaces such as submarines and aerospace shuttles [12] , [13] , [14] . In fact, in long-term space flight and submarine missions, CO 2 must be removed from the air and recycled because resupply opportunities are scarce. An average crew member requires approximately 0.84 kg of oxygen and emits approximately 1 kg of CO 2 per day [14] . Thus, the ability to continuously purify the exhaled air (with a maximum CO 2 concentration of 2–5%) will lead to an optimal recycling and considerable reduction in fresh air supply in remote confined spaces. Efficient CO 2 removal and resupply of fresh air is also critical in mining and rescue missions [15] , diving and most importantly in medical applications such as anaesthesia machines [16] . The use of anaesthesia machines is still a growing clinical trend worldwide, driven by the need to reduce cost and improve patient care via the use of efficient CO 2 sorbents. The CO 2 removal feature in anaesthesia machines is particularly important in semi-closed or closed rebreathing systems, as the rebreathing fraction is at least 50% of the exhaled gas volume, directed back to the patient after proper CO 2 removal in the next exhalation. Sodalime is currently the sorbent of choice in most commercially available anaesthesia machines. This sorbent exhibits a high CO 2 removal efficiency from exhaled air, with an average continuous operation of about 24 h using a prepacked commercial cartridge [17] . Nevertheless, a major drawback of this technology is that one sodalime cartridge can only be used for a single cycle and is non-recyclable, therefore generating undesirable waste as it should be disposed properly. Evidently, there is a pressing need to develop novel porous materials [18] that can adequately address the growing interest in low CO 2 concentration removal applications [10] . It is important to mention that only few materials were reported to efficiently adsorb traces of CO 2 , particularly with regards to DAC using a variety of amine-supported materials (for example, porous silica) [10] , [19] . Our quest for made-to-order materials that can address efficiently the separation and capture of trace CO 2 has prompted us to explore the potential of a burgeoning class of modular and tunable porous materials, namely metal-organic frameworks (MOFs), to tackle this ongoing challenge. Recently, MOFs were investigated intensively for intermediate and high CO 2 concentration removal applications such as post-combustion and precombustion capture, natural gas and biogas upgrading [20] , [21] , [22] , [23] . Nevertheless, the potential of MOFs to remove trace and low CO 2 concentration from gas streams was rarely debated [24] , [25] , [26] , [27] , [28] . The main reason for this lack of studies is that most of MOFs reported so far, with or without unsaturated metal centres or/and functionalized ligands, exhibit relatively low CO 2 uptake and selectivity particularly at relatively low CO 2 partial pressure. To overcome this downfall, various research groups have adopted the amine grafting chemistry and the acquired knowledge from amine-supported silica [19] , [22] as a prospective pathway to enhance the CO 2 adsorption energetics and uptake in MOFs and covalent organic frameworks [27] , [28] , [29] . Particularly, Jones and co-workers [28] reported for the first time the effect of ethylenediamine grafting on Mg-MOF-74 as a support for CO 2 adsorption from ultradilute gas streams such as ambient air. Correspondingly, Long and co-workers investigated the effect of N,N -dimethylethylenediamine grafting for DAC using an expanded isostructure of Mg-MOF-74 (ref. 27) [27] . Markedly, the few reported strategies targeting air capture using MOFs are centred on the aptitude of grafted amines to form a strong chemical bond (at least 70 kJ mol −1 ) with CO 2 , affording high affinity toward CO 2 and therefore high CO 2 selectivity. There is no reported study hitherto, to the best of our knowledge, on tuning the pore size of physical adsorption–based MOFs to target trace and low-concentration CO 2 removal. In this communication, we report how the reasoned choice of the appropriate MOF platform (here, SIFSIX -3-Cu material), characterized by suitable pore size, combined with the optimal CO 2 energetics (that is, strong, uniform and relatively low to allow reversible physical adsorption–desorption), is the key to target made-to-order porous materials for trace and low CO 2 concentration removal in general and DAC application in particular. Preparation and characterization of SIFSIX-3-Cu analogue The SIFSIX -3-Cu analogue was successfully prepared by layering a methanol solution of pyrazine in a glass tube onto a methanol solution of CuSiF 6 × H 2 O. On layering, an extremely fast formation of light violet powder was observed, which was left for 24 h in the mother solution. The powder was then collected and washed extensively with methanol then dried under vacuum and characterized using powder X-ray diffraction (PXRD). The PXRD diagram of SIFSIX -3-Cu analogue studied in this work was found not to match any related reported structures, that is, the Cu-2D structures or the 3D Zn analogue reported by Kita and co-workers [30] ( Supplementary Fig. 1 ). Despite extensive attempts, we were not able to isolate synthetic conditions affording single crystals of sufficient size suitable for single crystal diffraction studies and therefore structural determination by powder diffractometry was explored. The PXRD pattern of the crystalline powder, resulting from the reaction of CuSiF 6 × H 2 O with pyrazine in methanolic solution, was recorded on a high resolution PANalytical X’Pert MPD-PRO diffractometer with Cu–Kα radiation ( λ =1.5406 Å) in the range of 4 to 80° using a step of 0.05° (250 s per step). The indexation of the PXRD diagram, carried out using the McMaille software [30] , yielded a primitive orthorhombic cell ( M (20)=42.3 and F (20)=39.9 (0.0139, 36)). The cell parameters, a = b =6.919(1) Å, c =7.906(1) Å, were refined by a whole powder pattern fit using the Le Bail method [31] , implemented in the FULLPROF software [32] , and were consistent with those of the previously described SIFSIX -3-Zn. Hence, atomic positions of the latter were used as structure solution. The final Rietveld refinement permitted access to satisfactory results: R Bragg =0.051 and R Factor =0.056 ( Supplementary Fig. 2 ). 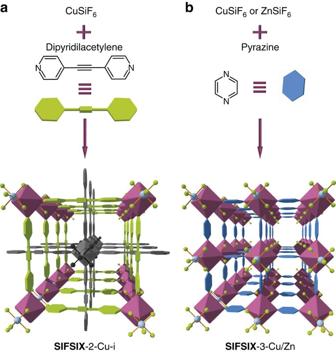Figure 1: Pore size tuning. Pore size tuning of the channel structures of (a)SIFSIX-2-Cu-i, (b)SIFSIX-3-Zn or/andSIFSIX-3-Cu. (a)SIFSIX-2-Cu-i; pores size 5.15 Å, Brunauer–Emmett–Teller (BET) apparent surface area (N2adsorption) 735 m2g−1. (b)SIFSIX-3-Zn; pores size 3.84 Å, BET apparent surface area 250 m2g−1(determined from the CO2adsorption isotherm at 298 K);SIFSIX-3-Cu; pores size 3.50 Å (NLDFT), BET and langmuir apparent surface area ca. 300 m2g−1(determined from the CO2adsorption isotherm at 298 K). Colour code: Dipyridylacetylene (dpa, thick light green polygon), pyrazine (pyz, blue polygon), Zn, Cu (purple polyhedra), Si (light blue spheres), F (light green spheres). All guest molecules are omitted for clarity. Note that the grey net represents the interpenetrated net inSIFSIX-2-Cu-i. The crystallographic data and refinement parameters of SIFSIX -3-Cu are summarized in Supplementary Table 1 . As initially expected, it is in very good agreement with the 3D structure of the Zn analogue reported previously ( Fig. 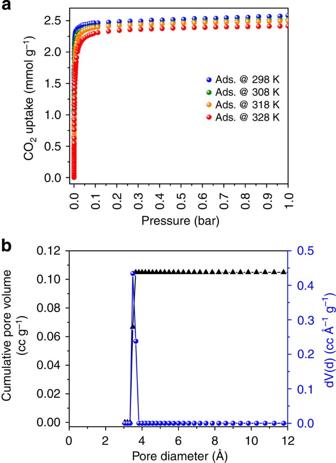Figure 2: CO2adsorption isotherms. CO2adsorption isotherms at variable temperatures forSIFSIX-3-Cu. TheSIFSIX-3-Cu analogue shows asteeper variable temperature adsorption isotherms at very low pressure indicative of strong CO2-SIFSIX-3-Cu interactions. (a) pore size distribution (PSD) derived from the CO2sorption isotherm (CO2at 273 K NLDFT) forSIFSIX-3-Cu. The PSD extracted from adsorption isotherms, shows an average pore size forSIFSIX-3-Cu centred at 3.5 Å(b). 1 ), but with a slightly smaller unit cell (378 versus 388 Å 3 ) attributed to the relatively stronger bonding between the Cu(II) and the pyrazine ( Supplementary Data 1 , Supplementary Table 2 ). The smaller unit cell of the Cu analogue is in good agreement with the relatively sharp pore size distribution analysis centred at 3.5 Å (average pore size), as determined from the CO 2 adsorption isotherms, using NLDFT model, which shows a smaller average pore size than the SIFSIX -3-Zn (3.5–4 Å) ( Fig. 2a ). The thermal gravimetric analysis of the SIFSIX -3-Cu showed a weight loss of about 10% for the dried sample in the range of 50–150 °C attributed to guest molecules ( Supplementary Fig. 3 ). Further gradual loss was observed above 150 °C and attributed to the framework decomposition. The thermal gravimetric analysis data for the SIFSIX -3-Cu is in a good agreement with the one reported for the SIFSIX -3-Zn analogue. Infrared spectrum for the SIFSIX -3-Cu ( Supplementary Fig. 4 ) exhibits bands characteristic of the C–H aromatic bonds associated to the pyrazine moiety at 3,114 and 3,073 cm −1 and bands characteristic for the C–N bond at 1,445, 1,122 and 1,070 cm −1 . Furthermore, the characteristic bands associated with the octahedral SiF 6 were also observed at 743 and 833 cm −1 (ref. 33 ). Figure 1: Pore size tuning. Pore size tuning of the channel structures of ( a ) SIFSIX -2-Cu-i, ( b ) SIFSIX -3-Zn or/and SIFSIX -3-Cu. ( a ) SIFSIX -2-Cu-i; pores size 5.15 Å, Brunauer–Emmett–Teller (BET) apparent surface area (N 2 adsorption) 735 m 2 g −1 . ( b ) SIFSIX -3-Zn; pores size 3.84 Å, BET apparent surface area 250 m 2 g −1 (determined from the CO 2 adsorption isotherm at 298 K); SIFSIX -3-Cu; pores size 3.50 Å (NLDFT), BET and langmuir apparent surface area ca. 300 m 2 g −1 (determined from the CO 2 adsorption isotherm at 298 K). Colour code: Dipyridylacetylene (dpa, thick light green polygon), pyrazine (pyz, blue polygon), Zn, Cu (purple polyhedra), Si (light blue spheres), F (light green spheres). All guest molecules are omitted for clarity. Note that the grey net represents the interpenetrated net in SIFSIX -2-Cu-i. Full size image Figure 2: CO 2 adsorption isotherms. CO 2 adsorption isotherms at variable temperatures for SIFSIX -3-Cu. The SIFSIX -3-Cu analogue shows asteeper variable temperature adsorption isotherms at very low pressure indicative of strong CO 2 - SIFSIX -3-Cu interactions. ( a ) pore size distribution (PSD) derived from the CO 2 sorption isotherm (CO 2 at 273 K NLDFT) for SIFSIX -3-Cu. The PSD extracted from adsorption isotherms, shows an average pore size for SIFSIX -3-Cu centred at 3.5 Å( b ). Full size image CO 2 adsorption studies In order to evaluate the potential of SIFSIX -3-Cu for CO 2 capture, we performed various CO 2 adsorption studies. It was our preconception that this new Cu analogue should at least show the same promising adsorption properties as the SIFSIX -3-Zn [23] . The Cu analogue shows even steeper variable temperature adsorption isotherms ( Fig. 2a ) at very low pressure indicative of relatively stronger CO 2 - SIFSIX -3-Cu interactions than the Zn analogue In order to further explore the possible sorption mechanistic behind this relatively enhanced uptake at low CO 2 loading, we explored the competitive adsorption kinetics of CO 2 /N 2 :10/90, CO 2 /CH 4 :50/50, CO 2 /H 2 :30/70 gas mixture adsorption ( Supplementary Fig. 5 ). As anticipated and based on similar studies carried out on the Zn analogue [23] , the uptake at equal times, including at equilibrium, for variable CO 2 compositions mixtures follows the behaviour of pure CO 2 . These findings suggest that similarly to the mechanistic suggested for SIFSIX -3-Zn, when CO 2 containing mixtures are in contact with SIFSIX -3-Cu, CO 2 adsorbs more strongly ( Supplementary Fig. 6 ) and rapidly than N 2 and by analogy also O 2 , CH 4 and H 2 ( Supplementary Fig. 5 ), thus occupying favourably most of the available space and adsorption sites and subsequently exclude other gases, a desirable feature in many CO 2 separation and purification applications. Interestingly, on the substitution of Zn by Cu, the Q st of CO 2 adsorption in the contracted structure increased by 20%, from 45 to 54 kJ mol −1 ( Fig. 3b ), in perfect agreement with the relatively steeper CO 2 adsorption isotherms in the case of the Cu analogue at very low pressure. 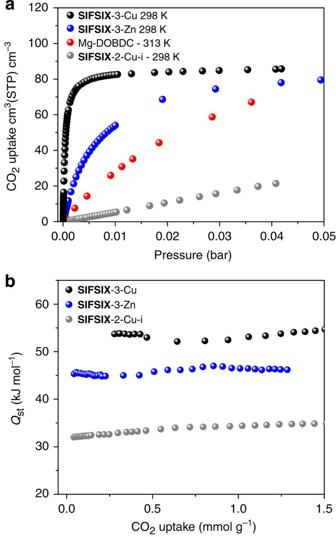Figure 3: CO2volumetric uptake. CO2volumetric uptake forSIFSIX-3-Cu at 298 K compared withSIFSIX-3-Zn,SIFSIX-2-Cu-I and Mg-MOF-74. The adsorption results at very low pressure (400 p.p.m.-5%) for theSIFSIX-3-Cu showed that the Cu analogue exhibits steeper adsorption isotherms at very low CO2concentration in comparison with other materials. At 7.6 torr (0.01 bar),SIFSIX-3-Cu uptakes 82.6 cm3(STP)/cm−3versus 55 and 28 cm3(STP)/cm−3forSIFSIX-3-Zn and Mg-MOF-74, respectively (a). Isosteric heats of adsorption at low coverage forSIFSIX-3-Cu,SIFSIX-3-Zn andSIFSIX-2-Cu-I. TheQstforSIFSIX-3-Cu was observed to be higher than the Zn analogue and steady constant up to relatively higher recorded CO2loadings. This is indicative of the presence of homogenous binding sites over the full range of CO2loading forSIFSIX-3-Cu (b). Figure 3: CO 2 volumetric uptake. CO 2 volumetric uptake for SIFSIX -3-Cu at 298 K compared with SIFSIX -3-Zn, SIFSIX -2-Cu-I and Mg-MOF-74. The adsorption results at very low pressure (400 p.p.m.-5%) for the SIFSIX -3-Cu showed that the Cu analogue exhibits steeper adsorption isotherms at very low CO 2 concentration in comparison with other materials. At 7.6 torr (0.01 bar), SIFSIX -3-Cu uptakes 82.6 cm 3 (STP)/cm −3 versus 55 and 28 cm 3 (STP)/cm −3 for SIFSIX -3-Zn and Mg-MOF-74, respectively ( a ). Isosteric heats of adsorption at low coverage for SIFSIX -3-Cu, SIFSIX -3-Zn and SIFSIX -2-Cu-I. The Q st for SIFSIX -3-Cu was observed to be higher than the Zn analogue and steady constant up to relatively higher recorded CO 2 loadings. This is indicative of the presence of homogenous binding sites over the full range of CO 2 loading for SIFSIX -3-Cu ( b ). Full size image Column breakthrough experiments Furthermore, the CO 2 selectivity for SIFSIX -3-Zn and SIFSIX -3-Cu was investigated experimentally at trace CO 2 using column breakthrough tests for binary CO 2 /N 2 : 1,000 p.p.m./99.9% mixture ( Fig. 4a ) at 298 K in dry as well as in humid conditions. The derived selectivity at breakthrough time (and not equilibrium) is intended to reflect the real selectivity in real processes. In a dry condition, the first CO 2 signal downstream the column was observed only after ca. 798 and ca. 1,922 min g −1 for SIFSIX -3-Zn and SIFSIX -3-Cu, respectively, after starting continuous CO 2 /N 2 gas mixture flux (5 cm 3 min −1 ), while N 2 breakthrough occurred immediately in few seconds. Accordingly, at 1,000 p.p.m. CO 2 and breakthrough time, SIFSIX -3-Cu shows higher selectivity (ca. 10500) than SIFSIX -3-Zn (7259). It is to mention that calculated and measured selectivity exceeding 1,000–2,000 are often subject to uncertainties associated with measurement of the gas uptake of weakly adsorbed gases (N 2 ; Supplementary Fig. 6 ) in the mixture, thus the reported selectivity is aimed mainly for relative comparison of the studied compounds in this work. In view of that, a direct comparison between the SIFSIX -3-Cu and the SIFSIX -3-Zn sorption properties show a 50% relative increase in CO 2 selectivity at 1,000 ppm CO 2 in a N 2 stream (ca. 10500 versus 7259). The steeper CO 2 signal after breakthrough for SIFSIX -3-Cu as compared with the Zn analogue is a direct indication of the steeper CO 2 adsorption for the Cu analogue as shown in Fig. 3a . 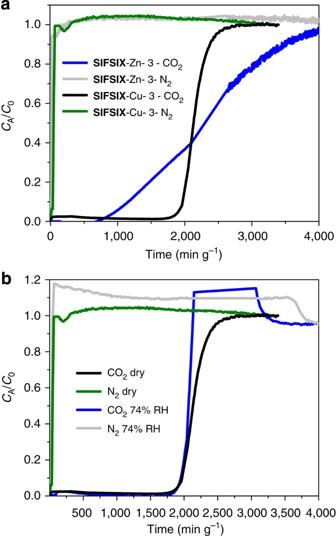Figure 4: Column breakthrough experiments. Column breakthrough test of CO2/N2:1,000 p.p.m./99.9% forSIFSIX-3-Cu,SIFSIX-3-Zn in dry condition (a). Column breakthrough test of CO2/N2:1,000 p.p.m./99.9% forSIFSIX-3-Cu in dry as well as at 74% RH (b). The CO2selectivity forSIFSIX-3-Zn andSIFSIX-3-Cu was investigated experimentally at trace CO2using column breakthrough tests for binary CO2/N2: 1,000 p.p.m./99.9% mixture at 298 K in dry as well as in humid conditions. In dry condition, the first CO2signal downstream the column was observed only after ca. 798 and ca. 1922, min g−1forSIFSIX-3-Zn andSIFSIX-3-Cu, respectively, after starting continuous CO2/N2gas mixture flux (5 cm3min−1), while N2breakthrough occurred immediately in few seconds. Figure 4: Column breakthrough experiments. Column breakthrough test of CO 2 /N 2 :1,000 p.p.m./99.9% for SIFSIX -3-Cu, SIFSIX -3-Zn in dry condition ( a ). Column breakthrough test of CO 2 /N 2 :1,000 p.p.m./99.9% for SIFSIX -3-Cu in dry as well as at 74% RH ( b ). The CO 2 selectivity for SIFSIX -3-Zn and SIFSIX -3-Cu was investigated experimentally at trace CO 2 using column breakthrough tests for binary CO 2 /N 2 : 1,000 p.p.m./99.9% mixture at 298 K in dry as well as in humid conditions. In dry condition, the first CO 2 signal downstream the column was observed only after ca. 798 and ca. 1922, min g −1 for SIFSIX -3-Zn and SIFSIX -3-Cu, respectively, after starting continuous CO 2 /N 2 gas mixture flux (5 cm 3 min −1 ), while N 2 breakthrough occurred immediately in few seconds. Full size image Recently, we reported CO 2 adsorption study on a series of isoreticular MOFs with periodically arrayed hexafluorosilicate ( SIFSIX ) pillars, called SIFSIX -2-Cu-i and SIFSIX -3-Zn ( Fig. 1 ) [23] . The aforementioned porous MOFs having a combination of tunable pore size (rather than large surface area) coupled with the requisite chemistry led to materials with uniformly aligned strong CO 2 adsorption sites and subsequently exhibiting a relatively fast and highly selective CO 2 behaviour over N 2 , CH 4 and H 2 (ref. 23 ). Particularly, the denser isoreticular analogue, namely SIFSIX -3-Zn, revealed steeper variable CO 2 adsorption isotherms ( Supplementary Fig. 7 ) than SIFSIX -2-Cu-i ( Supplementary Fig. 8 ). This material exhibits unique key features suitable for post-combustion capture (that is, the CO 2 partial pressure of 100 mbar), as well as precombustion capture (that is, high CO 2 concentration and high pressure). The pronounced steep CO 2 adsorption isotherms over a wide range of temperatures, particularly for this class of MOF materials, has inspired and compelled us to explore the potential of these SIFSIX MOFs for CO 2 adsorption in trace concentrations (that is, diluted streams in vacuum or in mixture containing a large fraction of N 2 up to 95%). In order to highlight the concealed potential of these MOFs for low CO 2 concentration applications (that is, involving CO 2 concentration below 5% or 50 mbar CO 2 partial pressure, such as anaesthesia machines and prepurification before air separation and air capture), single gas CO 2 adsorption properties were evaluated for SIFSIX -2-Cu-i and SIFSIX -3-Zn. Interestingly, the contraction of the pore size from 5.15 Å (for SIFSIX -2-Cu-i) to 3.84 Å (for SIFSIX -3-Zn) has prompted a drastic increase in CO 2 uptake ( Supplementary Fig. 9 ) and consequently a recorded highest CO 2 uptake ever reported for a given MOF in the range under 5% CO 2 . Specifically, SIFSIX -3-Zn showed an order of magnitude higher volumetric CO 2 uptake (55 cm 3 (STP)/cm 3 ) than to date best MOF materials such as Mg-MOF-74, (28 cm 3 (STP)/ cm 3 ) at 10 mbar (1% CO 2 ), while UTSA-16 (ref. 34) [34] , exhibits much lower CO 2 uptake similar to SIFSIX -2-Cu-i. The noticeable impact of pore size contraction on the adsorption energetics and uptake has impelled us to explore various pathways to further reduce the pore size of the SIFSIX -3-M derivative via metal substitution and evaluate its effect on the CO 2 adsorption properties. The rational is based on conventional coordination chemistry suggesting that replacement of Zn(II) by Cu(II) to form an isostructural SIFSIX -3-Cu will potentially induce an additional pore contraction due to Jahn–Teller distortions of the octahedral coordination geometry of Cu(II), CuN 4 F 2 . The Cu(II) has an open shell valence electron configuration 3d 9 , in contrast to Zn(II) with a close shell 3d 10 , and thus will experience a distorted octahedral coordination geometry with potentially elongated Cu–F (fluorine) bonds and relatively shorter Cu–N (nitrogen) bonds ( Supplementary Fig. 10 and Supplementary Table 2 ). Indeed, our analysis of readily available coordination polymers constructed from hexafluorosilicate ions with pyrazine supports our proposal and shows that the bonding of the Cu(II) with pyrazine leads to a slightly shorter M–N bond than the zinc analogue (see Supplementary Table 2 ) [35] . Accordingly, it is anticipated that successful substitution of Zn(II) by Cu(II) will permit access to the desired isostructural SIFSIX -3-Cu with relatively contracted pore size than the parent SIFSIX -3-Zn analogue and subsequent evaluation of its relative CO 2 adsorption properties. Examination of the SIFSIX -3-M adsorption results in the spectra of low-concentration applications (400 p.p.m.-5%) showed that the Cu analogue exhibits even steeper adsorption isotherms at very low CO 2 concentration ( Fig. 3a ) translated into the highest uptake ever reported for MOFs without unsaturated metal centres or exposed amino functionality at low CO 2 pressures below 38 torr (0.05 bar). This unprecedented finding is even more appealing owing to its fully physical adsorption nature where complete desorption of CO 2 was established under vacuum at only 323 K. At 7.6 torr (0.01 bar) SIFSIX -3-Cu uptakes 82.6 cm 3 (STP).cm −3 versus 55 and 28 cm 3 (STP).cm −3 for SIFSIX -3-Zn and Mg-MOF-74, respectively. Interestingly, the gravimetric uptake of SIFSIX -3-Cu at 400 p.p.m. and 298 K (1.24 mmol g −1 ) is ca. 10 and 15 times higher than the corresponding uptakes for SIFSIX -3-Zn (0.13 mmol g −1 ) and Mg-MOF-74 (0.08 mmol g −1 ) and even higher than the observed uptakes for most amine-supported silica materials (with optimal compromise of amine loading and kinetics) [22] at 298 K (for example TRI-PE-MCM-4 (1 mmol g −1 ) [10] , [22] ). Table 1 summarizes the CO 2 adsorption uptake at variable low CO 2 concentration (partial pressures) for SIFSIX compounds as compared with Mg-MOF-74 and amine-supported materials (including MOFs), relevant to different trace CO 2 removal applications. It is to notice that SIFSIX -3-Cu shows even higher CO 2 uptake at 400 p.p.m. and 328 K as compared with the corresponding uptake at 323 K for amine functionalized Mg-dobpdc-mmen ( Supplementary Table 3 ). Table 1 CO 2 adsorption uptake comparison. Full size table This increase is mainly attributed to the contracted pore size of the Cu analogue, which in turn (i) results in a relative increase of the charge density surrounding the adsorbed CO 2 molecules and (ii) favors the relatively faster CO 2 adsorption kinetics in comparison with N 2 . Indeed, the four flourine atoms pointing to the channel, in the same plane, are creating a proximal local charge density to the adsorbed CO 2 molecule, that is, the CO 2 –F average distance is much narrower in the case of the Cu analogue than the relatively open Zn analogue. It is suggested that the relatively narrower pore size allows and reinforces each CO 2 molecule to interact mutually with four fluorine centres, that is, the CO 2 molecule can interact potentially with four different surfaces of the square encompassing four fluorine adsorption sites at the same time. The Q st of CO 2 adsorption is an intrinsic property that dictates the affinity of the pore surface toward CO 2 ; this in turn plays a major role in determining the adsorption selectivity and the necessary energy to release CO 2 during the regeneration step. Although the Q st for CO 2 was slightly above the typical range of fully reversible CO 2 adsorption (30–50 kJ mol −1 ) [22] , SIFSIX -3-Cu was fully and promptly evacuated at 323 K in vacuum (or under N 2 flow environment). As in case of SIFSIX -3-Zn and SIFSIX -2-Cu-i, the Q st for CO 2 adsorption was steady constant up to relatively high CO 2 loadings indicating homogenous binding sites over the full range of CO 2 loading ( Fig. 3b )) [23] . The aforementioned competitive sorption kinetics of CO 2 /N 2 :10/90, CO 2 /CH 4 :50/50, CO 2 /H 2 :30/70 gas mixture adsorption experiments ( Supplementary Fig. 3 ) suggest a relatively high selective CO 2 adsorption that is plausible due to a synergistic interplay between CO 2 sorption thermodynamics and kinetics. This high selectivity was confirmed by performing prediction of CO 2 /N 2 gas mixture adsorption at equilibrium using Ideal Adsorption Solution Theory ( Supplementary Fig. 11 ). It is important to notice that the derived selectivity at breakthrough time is non-equilibrium data where, similarly to equilibrium Ideal Adsorption Solution Theory results, a complex interplay between strong electrostatic interactions and favourable kinetics toward CO 2 drive the high selectivity of CO 2 versus N 2 . The experimental results of the CO 2 /N 2 gas mixture adsorption testing in dry and humid conditions revealed that the CO 2 apparent selectivity at 1,000 p.p.m. CO 2 on SIFSIX -3-Cu was not affected by the presence of humidity as shown from the column breakthrough tests performed on both compounds at the relative humidity (RH) of 74% ( Fig. 4a ). This unprecedented finding was also valid in case of SIFSIX -3-Zn for the removal of low and higher CO 2 concentration [23] . Finally, as was demonstrated for SIFSIX -3-Zn, SIFSIX -3-Cu is a recyclable and moisture stable MOFs as inferred from the PXRD performed on associated samples after at least four cycles of CO 2 adsorption and breakthrough runs under dry and humid conditions (74% RH) ( Supplementary Fig. 12 ). In conclusion, we showed herein how a material design and engineering approach to pore size control in combination with suitable energetics of favourable electrostatics from an array of inorganic anions affords novel SIFSIX -3-Cu MOF with exceptional CO 2 uptake and selectivity in the context of air capture and trace CO 2 removal. This unique material exhibits very high CO 2 sorption energetics but fully reversible physical driven adsorption–desorption operations at very mild conditions, without the well-documented drawbacks associated with amine reactive chemistry. This work shows for the first time that MOFs, thanks to their ability for rational pore size modification and inorganic-organics moieties substitution, offer remarkable CO 2 physical adsorption attributes in highly diluted gas streams that other class of plain materials are unable to attain. Further work is underway to use the learning gained in the case of SIFSIX -3-M compounds to develop topologically and chemically different MOFs, aiming to target novel MOFs with suitable pore size and high charge density, for use in trace CO 2 , low and high concentration CO 2 removal. Preparation of SIFSIX-3-Cu A methanol solution (5.0 ml) of pyrazine (pyz, 0.30 g, 3.0 mmol) was layered in a glass tube onto a methanol solution (5.0 ml) of CuSiF 6 × H 2 O (0.325 g, 0.6 mmol). On layering, a fast formation of light violet powder was observed, and the powder was left for 24 h in the mother solution. The powder was then collected and washed extensively with methanol and then dried under vacuum. Characterization The PXRD patterns were recorded using a Panalytical X’pert PRO MPD X-ray Diffractometer with Cu Kα radiation ( λ =0.15418, nm, 45 kV, 40 mA). Low-pressure adsorption The low-pressure gas sorption isotherms were collected on Autosorb-1C (Quantachrome Instruments) Surface Area and Porosity Analyzer after activation of SIFSIX-3-Cu as follows. As-synthesized SIFSIX-3-Cu was exchanged with methanol for 3 days. The sample was degassed at room temperature under high vacuum (<5 μm Hg) for 12 h, then to 323 K for another 12 h before adsorption analysis. The apparent surface areas of SIFSIX-3-Cu were determined from the CO 2 adsorption isotherm collected at 298 K, respectively by applying the BET and Langmuir models. The determination of the isosteric heat of adsorption ( Q st ) for CO 2 was estimated by applying the Clausius–Clapeyron expression using the CO 2 adsorption isotherms measured at 298, 308, 318 and 328 K. The bath temperature was precisely controlled using a Julabo recirculating control system containing a mixture of ethylene glycol and water. Data points below 0.76 Torr were not used for this calculation, in order to avoid possible artifacts at very low coverage. Measurement of equilibrium and kinetics of adsorption Adsorption equilibrium measurements of pure gases were performed using a Rubotherm gravimetric–densimetric apparatus (Bochum, Germany) ( Supplementary Fig. 13 ), composed mainly of a magnetic suspension balance and a network of valves, mass flowmeters and temperature and pressure sensors. The magnetic suspension balance overcomes the disadvantages of other commercially available gravimetric instruments by separating the sensitive microbalance from the sample and the measuring atmosphere and is able to perform adsorption measurements across a wide pressure range, that is, from 0 to 20 MPa. The adsorption temperature may also be controlled within the range of 77 to 423 K. In a typical adsorption experiment, the adsorbent is precisely weighed and placed in a basket suspended by a permanent magnet through an electromagnet. The cell in which the basket is housed is then closed and vacuum or high pressure is applied. The gravimetric method allows the direct measurement of the reduced gas adsorbed amount Ω. Correction for the buoyancy effect is required to determine the excess and absolute adsorbed amount using equations 1 and 2, where V adsorbent and V ss and V adsorbed phase refer to the volume of the adsorbent, the volume of the suspension system and the volume of the adsorbed phase, respectively. The buoyancy effect resulted from the adsorbed phase maybe taken into account via correlation with the pore volume or with the theoretical density of the sample. Kinetic studies of CO 2 and CO 2 /N 2 :10/90 adsorption on SIFSIX -3-Cu was carried out using the Rubotherm gravimetric apparatus operating in dynamic regime. Initially, SIFSIX -3-Cu was properly evacuated at 323 K in vacuum. In order to achieve an immediate constancy of pressure (0.5 bar) during kinetics tests and avoid the often noisy uptake during the rapid introduction of the studied gas, an initial baseline was set-up using helium gas at 0.5 bar for single gases and 1 bar for mixture, then the studied single gas or mixture is flushed with a flow of 300 ml min −1 to avoid any dependence of the kinetics on the mass flow controller. Column breakthrough tests The experimental set-up used for dynamic breakthrough measurements is shown in Supplementary Fig. 13 . The gas manifold consisted of three lines fitted with mass flow controllers Line ‘A’ is used to feed an inert gas, most commonly helium, to activate the sample before each experiment. The other two lines, ‘B’ and ‘C’ feed a mixture of CO 2 and other gases like N 2 , CH 4 and H 2 . Hence, gas mixtures with concentrations representative of different industrial gases may be prepared. Whenever required, gases flowing through lines ‘B’ and ‘C’ may be mixed before entering a column packed with SIFSIX -3-Cu using a four-way valve. The stainless steel column was 27 mm in length with 4 mm of inner (6.4 mm outer) diameter. The column downstream was monitored using a Hiden analytical mass spectrometer. In a typical experiment, 0.1–0.4 g of adsorbent was treated at 298 K overnight under helium flow of 5 ml min −1 at 323 K, then the gas flow was switched to the desired gas mixture at the same flow rate. The complete breakthrough of CO 2 and other species was indicated by the downstream gas composition reaching that of the feed gas. Experiments in the presence of 74% RH were performed by flowing the gas mixture through water vapour saturator at 20 °C. The selectivity of CO 2 over N 2 is calculated using the equation below: How to cite this article: Shekhah, O. et al . Made-to-order metal-organic frameworks for trace carbon dioxide removal and air capture. Nat. Commun. 5:4228 doi: 10.1038/ncomms5228 (2014). Accession codes: The X-ray crystallographic data for structure reported in this article has been deposited at the Cambridge Crystallographic Data Centre (CCDC), under deposition number CCDC 970790. The data can be obtained free of charge from The Cambridge Crystallographic Data Center via www.ccdc.cam.ac.uk/data_request/cif .